Lactate racemase is a nickel-dependent enzyme activated by a widespread maturation system Racemases catalyse the inversion of stereochemistry in biological molecules, giving the organism the ability to use both isomers. Among them, lactate racemase remains unexplored due to its intrinsic instability and lack of molecular characterization. Here we determine the genetic basis of lactate racemization in Lactobacillus plantarum . We show that, unexpectedly, the racemase is a nickel-dependent enzyme with a novel α/β fold. In addition, we decipher the process leading to an active enzyme, which involves the activation of the apo-enzyme by a single nickel-containing maturation protein that requires preactivation by two other accessory proteins. Genomic investigations reveal the wide distribution of the lactate racemase system among prokaryotes, showing the high significance of both lactate enantiomers in carbon metabolism. The even broader distribution of the nickel-based maturation system suggests a function beyond activation of the lactate racemase and possibly linked with other undiscovered nickel-dependent enzymes. Lactic acid (L- and D-isomers) is an important and versatile compound produced by microbial fermentation. It is used in a range of applications in the agro-food, pharmaceutical and chemical sectors where optical purity is of tremendous importance [1] . Lactic acid is also common in numerous ecosystems and is involved in the energy metabolism of many prokaryotic species, as a product of sugar fermentation or as a carbon and electron source to sustain growth [2] . It can even be a component of the bacterial cell wall in order to confer resistance to the vancomycin antibiotic [3] , [4] . Micro-organisms have the remarkable ability to metabolize both lactic acid isomers via stereospecific lactate dehydrogenases. However, when only one stereospecific lactate dehydrogenase is present, production or utilization of the other isomer may proceed by lactate isomerization involving a specific lactate racemase (Lar) [5] . This activity was first reported in Clostridium beijerinckii (formerly C. butylicum ) [6] and, since then, it has been identified in several species including lactobacilli [7] , [8] , [9] , [10] . Besides Lar, the only known α-hydroxyacid racemase is the mandelate racemase, which is a Mg-dependent enzyme of the enolase superfamily [11] . The majority of racemases are amino acid racemases, which are either pyridoxal 5′-phosphate (PLP)-dependent or PLP-independent enzymes [12] . Both mandelate racemase and PLP-independent racemases rely on intramolecular stabilization of a deprotonated reaction intermediate for their catalysis [11] , [13] . Concerning the Lar, another mechanism is probably taking place due to the absence of an electron-withdrawing group on lactate. A few reports have addressed the Lar activity of Lactobacillus sakei , C. beijerinckii and C. acetobutylicum and suggested a hydride transfer mechanism [14] , [15] , [16] , [17] . However, the Lar enzymes were not identified in these species. In Lactobacillus plantarum , we previously identified a gene cluster, named lar , which is positively regulated by L-lactate and is required for lactate racemization [4] . In this species, we have shown that D-lactate is an essential compound of the cell wall peptidoglycan and have proposed that the Lar acts as a rescue enzyme to ensure D-lactate production in physiological conditions where its production by the D-lactate dehydrogenase is not sufficient [4] . The identified lar locus responsible for lactate racemization is composed of five genes that are organized in an operon: larA , larB , larC , larD and larE . Except for the larD gene, encoding a lactic acid transporter shown recently to increase the rate of lactate racemization in vivo [18] , the role of the other Lar proteins in the racemization of lactate could not be defined [4] . No similarity to any protein of known structure or function could be found for LarA and LarC. As for LarB and LarE, although similar proteins were found, the resulting predictions were not very informative: LarE was predicted as an ATP-utilizing enzyme of the PP-loop superfamily, and part of the C-terminal sequence of LarB was found to be similar to N 5 -carboxyaminoimidazole ribonucleotide mutase [4] . In this study, we report the first molecular and structural characterization of a Lar, a unique racemase that uses nickel as an essential cofactor. By a combination of in vivo and in vitro experiments, we demonstrate that the Lar is activated by a novel maturation system composed of three accessory proteins that are essential for nickel delivery in the active site of the apo-enzyme. Using in silico analyses, we reveal the widespread distribution of this new nickel-based maturation system among prokaryotes, suggesting an important role not only for lactate metabolism but potentially also for the activation of other Ni-dependent enzymes. Four proteins and Ni are required for in vivo Lar activity In order to investigate whether the previously identified larA–E operon of L. plantarum [4] is sufficient to confer Lar activity, it was cloned on a multicopy plasmid and expressed in the heterologous host Lactococcus lactis —a lactic acid bacterium with no Lar activity—under the control of a nisin-inducible promoter. Although Lar proteins could easily be detected from cell extracts of nisin-induced cultures after gel separation, no Lar activity could be measured. As the larA–E operon was not sufficient to confer Lar activity, we hypothesized that additional genes were required. To obtain an extended view of potential L. plantarum genes involved in lactate racemization, a transcriptomic approach was used based on the induction of Lar activity by L-lactate but not by DL-lactate [4] . 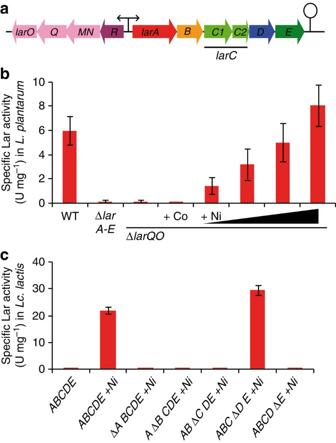Figure 1: Analysis of thelargene cluster and its encoded Lar proteins. (a)larlocus ofL. plantarumwith the two operonslarR(MN)QOandlarA–E. (b) Effect oflarA–EandlarQOdeletions inL. plantarumon specific Lar activity in crude extracts. Supplementation assays of the ΔlarQOmutant with CoCl2(1 mM) and NiCl2(0.2, 0.4, 0.8 and 1.5 mM). (c) Specific Lar activity in crude extracts after the expression oflargenes inLc. lactis:larA–Eoperon ±NiCl2(1 mM), in frame deletions of individual genes (Δ) in thelarA–Eoperon with NiCl2supplementation (1 mM). Data inbandcare average of quadruplicates from one representative experiment of three independent experiments showing similar results. The error bars represent the 95% confidence interval (Student’st-test). Besides the previously reported larA–E operon [4] , we identified a second operon consisting of four genes ( lp_0103 to lp_0100 ) as positively induced by L-lactate ( Supplementary Table 1 ). This operon is located upstream of the larA–E operon in an opposite orientation ( Fig. 1a ). The first gene of the operon, named larR , codes for a transcriptional regulator of the Crp-Fnr family while the other three genes, lar ( MN ) QO , encode a three-component ATP-binding cassette (ABC) transporter ( Fig. 1a ). Intriguingly, this ABC transporter is homologous to high-affinity Ni transporters, which are generally associated with Ni-dependent enzymes, although no such enzyme is known or predicted in L. plantarum [19] . We investigated the contribution of this transporter to the Lar activity by marker-less gene inactivation. Deletion of larQO resulted in the same Lar-deficient phenotype as was observed in the larA–E deletion mutant strain ( Fig. 1b ). Complementation of this phenotype was attempted through supplementation of the culture medium with Co(II), Ni(II) and other divalent metals. Among all tested supplements, only Ni(II) was able to restore Lar activity in the Δ larQO mutant. This Ni(II)-dependent recovery of Lar activity was dose-dependent and a full recovery of the wild-type activity was achieved with 1.5 mM Ni(II) ( Fig. 1b ). To validate the importance of nickel as an essential cofactor for Lar activity, the culture medium of the Lc. lactis strain overexpressing the larA–E operon was supplemented with Ni(II). Notably, the presence of nickel resulted in the observation of Lar activity at a level three- to fourfold higher than in L. plantarum ( Fig. 1c ). These results show that the transfer of the Lar activity of L. plantarum in this heterologous host only relies on the expression of the larA–E operon as long as Ni is supplemented to the growth medium. Figure 1: Analysis of the lar gene cluster and its encoded Lar proteins. ( a ) lar locus of L. plantarum with the two operons larR ( MN ) QO and larA–E . ( b ) Effect of larA–E and larQO deletions in L. plantarum on specific Lar activity in crude extracts. Supplementation assays of the Δ larQO mutant with CoCl 2 (1 mM) and NiCl 2 (0.2, 0.4, 0.8 and 1.5 mM). ( c ) Specific Lar activity in crude extracts after the expression of lar genes in Lc. lactis : larA–E operon ±NiCl 2 (1 mM), in frame deletions of individual genes (Δ) in the larA–E operon with NiCl 2 supplementation (1 mM). Data in b and c are average of quadruplicates from one representative experiment of three independent experiments showing similar results. The error bars represent the 95% confidence interval (Student’s t -test). Full size image We then addressed the question of the contribution of individual lar genes to Lar activity. For this, each gene of the larA–E operon was deleted from the overexpression plasmid and the Lar activity was assayed in Lc. lactis . Of the five genes of the operon, four were strictly required for Lar activity, while the lactic acid transporter encoding gene ( larD ) was dispensable ( Fig. 1c ). This in vivo investigation revealed that lactate racemization was surprisingly dependent on the presence of four proteins and requires the unusual nickel cofactor. This metal was demonstrated as an essential cofactor for only eight enzymes, all belonging to the family of Ni-dependent metalloenzymes [20] . LarA is the Ni-dependent Lar To evaluate which protein is catalytically active as Lar, each protein of the operon was purified in the presence of Ni in the culture medium. For purification needs, each one was individually fused to a StrepII-tag at either its N- or C terminus and expressed in Lc. lactis using the larA–E expression vector. Compatibility of the inserted StrepII-tags with Lar activity was verified before purification ( Fig. 2a ). Purification of LarA and LarE could readily be achieved from the strain expressing the entire operon, whereas tagged LarB and LarC could only be purified when the corresponding genes were individually subcloned (LarA Lp , LarB, larC and LarE; Fig. 2b ). For crystallographic needs, we also purified a LarA ortholog from a thermophilic bacterium, Thermoanaerobacterium thermosaccharolyticum , which shows 53% sequence identity with LarA Lp and also racemizes lactate when purified from cells expressing an artificial operon containing the larBCE genes from L. plantarum (LarA Tt ; Fig. 2a,b ). 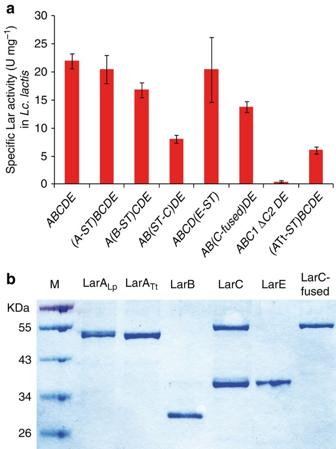Figure 2: StrepII-tag insertions in thelarA–Eoperon and LarC modifications. (a) Specific Lar activity ofLc. lactisstrains expressing the entirelarA–Eoperon ofL. plantarum(ABCDE) in which one of the Lar proteins has been fused to a StrepII-tag at either the N- (ST-X) or C terminus (X-ST), harbouring a 1-bp insertion at the end oflarC1(C-fused), with the in frame deletions oflarC2(ΔC2) and expressing the artificial operonlarATtBCDEin which LarATthas been fused to a StrepII-tag at the C terminus (ATt-ST). NiCl2was added in all cases (1 mM). Data are average of quadruplicates from one representative experiment of two independent experiments showing similar results. The error bars represent the 95% confidence interval (Student’st-test). (b) SDS-PAGE of purified StrepII-tagged LarALp, LarATt, LarB, LarC (LarC1 and LarC1C2), LarE and LarC-fused (only LarC1C2). The identity of each purified Lar protein was confirmed by MALDI-TOF (matrix-assisted laser desorption/ionisation–time-of-flight mass spectrometry) analysis ( Supplementary Table 2 ). Upon purification of StrepII-tagged LarC, two distinct proteins were observed with molecular masses of ~36 and 55 kDa ( Fig. 2b ). The small protein corresponded to the protein encoded by the larC1 open reading frame (ORF) alone (LarC1). The protein showing a higher molecular mass was found to be a fusion between the proteins encoded by the larC1 and larC2 ORFs (LarC), most likely resulting from a programmed ribosomal frameshift [21] . In agreement, artificial in-frame fusion between larC1 and larC2 ORFs resulted in the expression of only the full-length LarC protein, which did not affect Lar activity ( Fig. 2a,b ). Conversely, expression of LarC1 alone resulted in a complete loss of Lar activity ( Fig. 2a ). Together, these results show that LarC is the functional form of the protein. Figure 2: StrepII-tag insertions in the larA–E operon and LarC modifications. ( a ) Specific Lar activity of Lc. lactis strains expressing the entire larA–E operon of L. plantarum (ABCDE) in which one of the Lar proteins has been fused to a StrepII-tag at either the N- (ST-X) or C terminus (X-ST), harbouring a 1-bp insertion at the end of larC1 (C-fused), with the in frame deletions of larC2 (ΔC2) and expressing the artificial operon larA Tt BCDE in which LarA Tt has been fused to a StrepII-tag at the C terminus (A Tt -ST). NiCl 2 was added in all cases (1 mM). Data are average of quadruplicates from one representative experiment of two independent experiments showing similar results. The error bars represent the 95% confidence interval (Student’s t -test). ( b ) SDS-PAGE of purified StrepII-tagged LarA Lp , LarA Tt , LarB, LarC (LarC1 and LarC1C2), LarE and LarC-fused (only LarC1C2). Full size image Of the four purified L. plantarum proteins, LarA was the only one capable of catalysing lactate racemization (LarA Lp and LarA Tt ; Table 1 and Supplementary Fig. 1 ). The Ni content of both purified LarA homologues was assayed by inductively coupled plasma atomic emission spectroscopy (ICP-AES) and visible spectroscopy using a chromogenic chelator (4-(2-pyridylazo)resorcinol (PAR)) [22] . Purified LarA homologues contained ~0.1–0.2 mol Ni per mol of protein ( Table 1 ). Upon incubation at room temperature, free Ni became progressively available, which was correlated with a progressive loss of activity ( Supplementary Fig. 2a ), indicating that Ni was leaking out of LarA. This loss of activity could be delayed, but not prevented, by the addition of NiCl 2 or L-ascorbic acid in the buffer ( Supplementary Fig. 2b ). These observations confirm the previously reported protection of Lar activity by reducing agents (L-ascorbic acid, dithioerythritol and β-mercaptoethanol) [7] and further highlight Ni leakage as an inactivation consequence. The kinetic parameters of both LarA homologues were also determined ( Table 1 and Supplementary Fig. 1 ). Albeit in the millimolar range, the K m values determined for LarA Lp are still significantly lower than the cytoplasmic lactate concentration in L. plantarum (>200 mM) [23] , and in the range of previously determined values for the Lar of L. sakei [14] . Given the partial Ni loading of purified LarA, its rate constants are more probably underestimated by at least fivefold. Altogether, these results show that LarA is the Ni-dependent Lar and suggest that the other Lar proteins act as accessory proteins for LarA activation. Maturation proteins are similarly reported for the activation of three other nickel-dependent enzymes [24] . Table 1 Properties of LarA from L. plantarum (LarA Lp ) and T. thermosaccharolyticum (LarA Tt ). Full size table LarA shows a novel α/β fold In order to identify the Lar catalytic site, the crystal structure of LarA Tt was determined. LarA Tt crystals were obtained after 2 months of crystallization. The structure was solved by multi-wavelength anomalous dispersion and the structure was refined to 1.8 Å ( Table 2 ). As expected, given the spontaneous Ni leakage from the enzyme, no Ni was present in the crystals. Crystals were soaked with NiCl 2 in presence or absence of lactate but no Ni incorporation was observed. The enzyme crystallized as a dimer with both monomers showing nearly identical structures ( Fig. 3a ). LarA contains 18 β-strands and 16 α-helices arranged in a novel fold composed of two domains of similar size, connected by two hinges ( Fig. 3b and Supplementary Fig. 3 for a stereo view). As the strand order 162345, observed in domain A, was not found in any fold of the SCOP database [25] , we hypothesize that LarA shows a new fold of the α/β class. Table 2 Data collection and refinement statistics of LarA Tt . 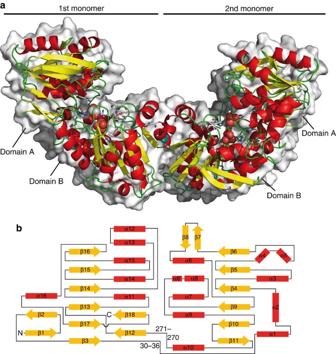Figure 3: 3D structure and topology of LarA. (a) 3D dimeric structure of LarATt(RSCB Protein Data Bank (PDB) accession code 2YJG). α-Helices are in red, β-sheets in yellow, and loops in green. Conserved residues are shown in stick representation and ethylene glycol, sulphate and Mg(II) are in sphere representation with C in white, N in blue, O in red, Mg in cyan and S in yellow. Surface representation is shown at the background. (b) The Lar fold. α-Helices are in red, β-strands in yellow and loops are in black. The topology of the β-sheet of domain A is six parallel β-strands in the order 162345. The topology of the β-sheet of domain B is six β-strands in the order 321456 with the last β-strand antiparallel to the rest. The numbers indicate the position of the two hinges. Full size table Figure 3: 3D structure and topology of LarA. ( a ) 3D dimeric structure of LarA Tt (RSCB Protein Data Bank (PDB) accession code 2YJG). α-Helices are in red, β-sheets in yellow, and loops in green. Conserved residues are shown in stick representation and ethylene glycol, sulphate and Mg(II) are in sphere representation with C in white, N in blue, O in red, Mg in cyan and S in yellow. Surface representation is shown at the background. ( b ) The Lar fold. α-Helices are in red, β-strands in yellow and loops are in black. The topology of the β-sheet of domain A is six parallel β-strands in the order 162345. The topology of the β-sheet of domain B is six β-strands in the order 321456 with the last β-strand antiparallel to the rest. The numbers indicate the position of the two hinges. Full size image Comparison of 148 LarA homologues shows that 16 residues (3 His, 9 Gly, 2 Lys, 1 Asp and 1 Arg) are fully conserved ( Supplementary Figs 4 and 5 for a representative alignment of 10 LarA homologues from remote species). These residues are located at the interface between the two domains, most of them belonging to domain B ( Fig. 4 ). Although the crystals were obtained in the absence of substrate (lactate) or inhibitor, sulphate and ethylene glycol were present during crystallization, and appear to form hydrogen bonds with conserved residues (His 108, His 200, K184, K298 and R75; Fig. 4a,b and Supplementary Fig. 6 ). The O-C-C-O atom connectivity of ethylene glycol is also found in lactate, suggesting that the molecule occupies the substrate-binding site. These observations suggest that the conserved residues at the interface between the two domains constitute the catalytic site. 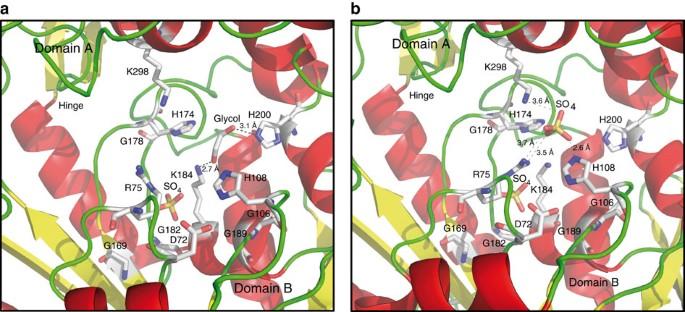Figure 4: LarA catalytic site. (a) Catalytic site of the first monomer (b) Catalytic site of the second monomer. Sulphates and ethylene glycol are displayed. Colour code as inFig. 3a. Figure 4: LarA catalytic site. ( a ) Catalytic site of the first monomer ( b ) Catalytic site of the second monomer. Sulphates and ethylene glycol are displayed. Colour code as in Fig. 3a . Full size image LarA Ni centre is coordinated by His residues In order to characterize the binding site of Ni in the LarA structure, X-ray absorption spectroscopy (XAS) experiments were conducted on frozen samples of purified LarA Lp and LarA Tt . The two LarA homologues show similar pre-edge XANES (X-ray absorption near edge structure) features that consist of 1s to 3d (8,332.5 eV) and 1s to 4p (8,337.2 eV) transitions ( Fig. 5a ). These two transitions are consistent with either a four-coordinate square planar nickel centre or a five coordinate square pyramidal site [26] , the latter being favored due to the well-defined shape of the 1s to 3d transition ( Fig. 5a ). LarA was also analysed by EXAFS (extended X-ray absorption fine structure). The Fourier-transformed spectra (FT) of LarA Tt ( Fig. 5b,c ) is dominated by an intense feature at 1.7 Å with a smaller peak at 1.2 Å, suggesting the presence of a split first scattering shell. The goodness of fit (%R) from single scattering fits ( Supplementary Table 3 ) improves significantly with splitting of the first scattering shell and addition of contributions from sulphur-scattering atoms. These preliminary fits point to a five-coordinated nickel centre dominated by N/O scatterers (N) and complemented by a single S/Cl scatterer (S). The Fourier-transformed spectra also show density between 2.5 Å to 4.0 Å of R-space, consistent with multiple scattering ligands, generally attributed to the presence of His residues in biological samples. Although the EXAFS data forms a complicated fitting picture, fits consisting of multiple (2–3) His residues (H) are generally favored and needed to account for the density. Physically meaningful fits were only achieved when the histidine scattering shells were split. The fits converged on three models, two five-coordinate fits (N1H2H1S1 and N2H1H1S1) and a six-coordinate fit (N2H2H1S1), which were statistically similar ( Supplementary Table 3 ), but the XANES analysis reported above supports the five-coordinate fit. The prediction can be further refined when glycerol (G) is taken into consideration, the latter is an additive in the buffer and also features the O-C-C-O atom connectivity found into lactate ( Fig. 5c and Supplementary Table 3 ). These results indicate that the conserved His residues (H174, H200 or H108), which are located in the supposed catalytic site, and glycerol (or a similar molecule) may coordinate nickel in LarA. 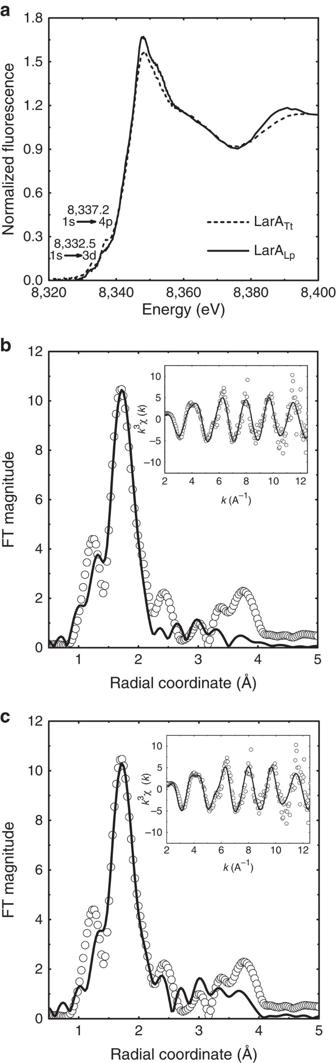Figure 5: XANES and EXAFS spectra. (a) Ni K-edge XANES spectra of LarATtand LarALpshowing a four-square planar or five-square pyramidal coordination geometry for nickel binding; 10 mM Tris buffer, pH 7.5, 20% glycerol. (b) Ni K-edge EXAFS spectra of LarATtand fit for N2H1H1S1. Fourier-transformed EXAFS spectra (no phase correction, FT window=2–12.5 Å−1). Inset: k3-weighted unfiltered EXAFS spectra; data (circles), best fit (line). (c) Ni K-edge EXAFS spectra of LarATtand fit for GH2H1S1. Fourier-transformed EXAFS spectra (no phase correction, FT window=2–12.5 Å−1). Inset: k3-weighted unfiltered EXAFS spectra; data (circles), best fit (line). N: N/O scatterers, H: histidine scatterer, S: S/Cl scatterers and G: glycerol scatterer. Figure 5: XANES and EXAFS spectra. ( a ) Ni K-edge XANES spectra of LarA Tt and LarA Lp showing a four-square planar or five-square pyramidal coordination geometry for nickel binding; 10 mM Tris buffer, pH 7.5, 20% glycerol. ( b ) Ni K-edge EXAFS spectra of LarA Tt and fit for N2H1H1S1. Fourier-transformed EXAFS spectra (no phase correction, FT window=2–12.5 Å −1 ). Inset: k 3 -weighted unfiltered EXAFS spectra; data (circles), best fit (line). ( c ) Ni K-edge EXAFS spectra of LarA Tt and fit for GH2H1S1. Fourier-transformed EXAFS spectra (no phase correction, FT window=2–12.5 Å −1 ). Inset: k 3 -weighted unfiltered EXAFS spectra; data (circles), best fit (line). N: N/O scatterers, H: histidine scatterer, S: S/Cl scatterers and G: glycerol scatterer. Full size image LarC and LarE are Ni-containing proteins The assembly of nickel metallocenters by maturases usually requires the presence of at least one nickel carrier (for example, UreE in the urease system) that inserts Ni into the catalytic site [24] . Therefore, Ni was assayed in purified LarB, LarC and LarE by ICP-AES and visible spectroscopy using PAR ( Fig. 6a ) [22] . Ni was detected in LarC and LarE, albeit at different levels. Purified LarC displayed the highest Ni content among all Lar proteins with 7–10 mol Ni per mol of protein, considering that purified LarC is a mixture of LarC1 and LarC in a ratio of about 1.5:1 ( Fig. 2b ). This observation is consistent with the strong over-representation of His residues in LarC1 (8.0 versus 1.7% in average L. plantarum proteins [27] ) and the presence of a His-rich region. As for LarE, 0.8 mol Ni per mol of protein were found when the protein was expressed in the presence of Ni and LarBC. The amount of Ni decreased to 0.08 mol Ni per mol of protein when no Ni(II) was present in the culture medium during LarE expression, and went further down to undetectable levels when Ni(II) was present but LarBC were not co-expressed ( Fig. 6a ). This shows the requirement of LarC and/or LarB for the Ni loading of LarE, the Ni probably being provided by LarC that could act as a Ni carrier/storage protein. 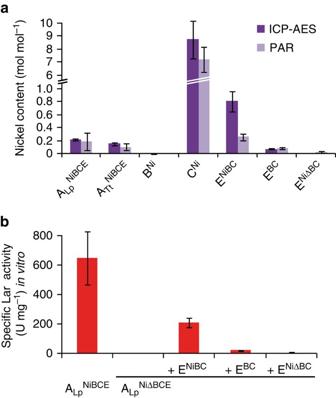Figure 6: Lar accessory proteins. (a) Ni content of Lar proteins as measured by PAR assays and ICP-AES. PAR data are average of two independent experiments (triplicates in each experiment). ICP-AES data are average of duplicates from one experiment. (b) Specific Lar activity of purified proteins andin vitroactivation of apo-LarA. ALpNiBCE, LarA purified from aLc. lactisstrain expressing LarBCE and cultivated in the presence of Ni(II); ALpNiΔBCE, LarA purified from aLc. lactisstrain not expressing LarBCE and cultivated in the presence of Ni(II); +ENiBC, assay performed in the presence of an excess of LarE purified from aLc. lactisstrain expressing LarBC and cultivated in the presence of Ni(II); +EBC, assay performed in the presence of an excess of LarE purified from aLc. lactisstrain expressing LarBC and cultivated in the absence of Ni(II); +ENiΔBC, assay performed in the presence of an excess of LarE purified from aLc. lactisstrain not expressing LarBC and cultivated in the presence of Ni(II); BNi, LarB purified from aLc. lactisstrain cultivated in the presence of Ni(II); and CNi, LarC purified from aLc. lactisstrain cultivated in the presence of Ni(II). Data are average of quadruplicates from one representative experiment of two independent experiments showing similar results. L-lactate was used as a substrate for all Lar activity measurements. The error bars represent the 95% confidence interval (Student’st-test) inaandb. Figure 6: Lar accessory proteins. ( a ) Ni content of Lar proteins as measured by PAR assays and ICP-AES. PAR data are average of two independent experiments (triplicates in each experiment). ICP-AES data are average of duplicates from one experiment. ( b ) Specific Lar activity of purified proteins and in vitro activation of apo-LarA. A Lp NiBCE , LarA purified from a Lc. lactis strain expressing LarBCE and cultivated in the presence of Ni(II); A Lp NiΔBCE , LarA purified from a Lc. lactis strain not expressing LarBCE and cultivated in the presence of Ni(II); +E NiBC , assay performed in the presence of an excess of LarE purified from a Lc. lactis strain expressing LarBC and cultivated in the presence of Ni(II); +E BC , assay performed in the presence of an excess of LarE purified from a Lc. lactis strain expressing LarBC and cultivated in the absence of Ni(II); +E NiΔBC , assay performed in the presence of an excess of LarE purified from a Lc. lactis strain not expressing LarBC and cultivated in the presence of Ni(II); B Ni , LarB purified from a Lc. lactis strain cultivated in the presence of Ni(II); and C Ni , LarC purified from a Lc. lactis strain cultivated in the presence of Ni(II). Data are average of quadruplicates from one representative experiment of two independent experiments showing similar results. L-lactate was used as a substrate for all Lar activity measurements. The error bars represent the 95% confidence interval (Student’s t -test) in a and b . Full size image In vitro activation of LarA by a LarBC-activated LarE To investigate LarA activation by the putative Lar accessory proteins, in vitro experiments were performed. For this purpose, an inactive version of LarA (apoprotein, apo-LarA) was purified from a strain lacking larBCE (A Lp NiΔBCE ; Fig. 6b ).The ability of purified LarB, LarC and LarE to activate apo-LarA was then evaluated in various combinations and in the presence of different cofactors known to activate other Ni-dependent enzymes ( Supplementary Table 4 ). Notably, apo-LarA could be readily activated by adding purified LarE, but only if LarE was co-expressed with LarB and LarC and in the presence of Ni(II) (LarE NiBC , Fig. 6b ). No additional cofactor was required for this activation or shown to enhance apo-LarA activation by LarE ( Supplementary Table 4 ). These in vitro results demonstrate that Ni-loaded LarE acts as a maturation protein responsible for the activation of apo-LarA, and indicate that LarB and LarC are involved in the activation of LarE before apo-LarA activation. LarA and its maturation system are widespread in prokaryotes In order to get an overview of the role of Lar proteins in the microbial world, we analysed the distribution of lar genes from the larA–E operon in prokaryotic genomes. The lar genes encoding putative nickel transport and regulation proteins (cluster larR ( MN ) QO ) were not considered in this in silico analysis since nickel transport may be achieved by a wide variety of transporters [19] and transcriptional regulation of lactate racemization is not a prerequisite for this function. BlastP searches were performed against all complete prokaryotic genomes of the NCBI database (1,087 bacterial and archaeal genomes) using the different Lar proteins of L. plantarum WCFS1 as query sequences. This search revealed the presence of at least one homologue of larA , larB , larC , larD and larE , in 111, 260, 263, 9 and 259 species, respectively ( Fig. 7a ). The larA gene appears to be present in most bacterial classes and in archaea. The largest number of larA homologues were found in clostridia (26 out of 78 species) and in δ proteobacteria (19 out of 39 species), some species bearing up to 4 larA paralogues ( Supplementary Tables 5, 6 and 7 ). This suggests that lactate racemization may not only be useful to lactic acid producers such as lactic acid bacteria but also to a wide variety of species with different metabolisms, including acetogenic, sulphate-reducing, metal-reducing, fumarate-reducing and butyrate-producing bacteria ( Supplementary Table 6 ). These bacterial taxons are indeed documented to utilize lactate as a carbon and/or electron source [28] , [29] , [30] , [31] . 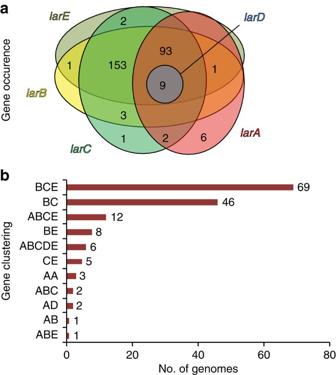Figure 7:In silicoanalysis oflargenes. (a) Distribution of thelargenes in 1,087 sequenced bacterial and archaeal genomes. The Venn diagram illustrates the occurrence and overlap of predictedlarA(red),larB(yellow),larC(green),larD(blue) andlarEgenes (olive green). (b) Gene clustering of predictedlarA(A),larB(B),larC(C),larD(D) andlarE(E) genes in 1,087 bacterial and archaeal genomes. The numbers indicate the total number of clusters of each type. Non-clustered representatives are not included inb. Figure 7: In silico analysis of lar genes. ( a ) Distribution of the lar genes in 1,087 sequenced bacterial and archaeal genomes. The Venn diagram illustrates the occurrence and overlap of predicted larA (red), larB (yellow), larC (green), larD (blue) and larE genes (olive green). ( b ) Gene clustering of predicted larA (A), larB (B), larC (C), larD (D) and larE (E) genes in 1,087 bacterial and archaeal genomes. The numbers indicate the total number of clusters of each type. Non-clustered representatives are not included in b . Full size image Ninety-two per cent of the genomes bearing a larA homologue (102 out of 111 genomes) also contained the genes for the Lar accessory proteins ( larBCE ), further reinforcing the necessity of these proteins for LarA activation ( Fig. 7a ). Strikingly, the accessory protein-encoding genes were also found in 153 species with no larA homologues ( Fig. 7a ). To get a better view of the relationship between these genes, their clustering within each genome was examined ( Fig. 7b ). The presence of a complete cluster including larABCDE seems to be restricted to only six species, all of them belonging to the lactobacillaceae family ( Supplementary Table 6 ). As LarD was shown to be a lactic acid channel [18] , the expression of the whole cluster is expected to enhance the lactic acid transport, besides the racemization of lactate. Twelve species harbour a larABCE cluster, but the most recurrent cluster only includes larBCE , which appears in 69 species, among which only 23 species also possess a larA homologue ( Fig. 7b ). Such putative operonic structures suggest that these genes likely participate in a common function that is not necessarily linked with lactate racemization. Nickel is an essential component of eight metalloenzymes involved in energy (for example, hydrogenases) and nitrogen (urease) metabolism and is used by 80% of the archaea and 60% of the eubacteria [32] . As we showed that the Lar is Ni-dependent, the number of Ni enzymes is now brought to nine [20] . In this study, we characterized the Lar, LarA, and determined its 3D structure, which shows a novel multidomain fold of the α/β class. 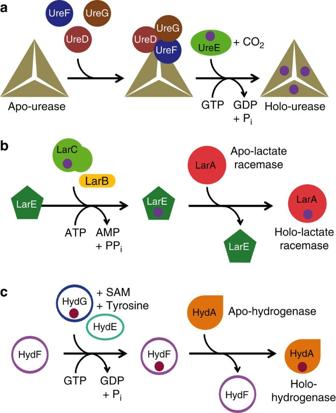Figure 8: Model of assembly of Lar metallocenter. (a) Assembly of urease metallocenter; one triangle represents one urease trimer of UreABC. UreD, UreE, UreF and UreG are the urease accessory proteins. (b) Proposed model for the assembly of Lar metallocenter. LarA is the Lar, while LarB, LarC and LarE are the Lar accessory proteins. (c) Assembly of [FeFe]-hydrogenase metallocenter. HydA is the [FeFe]-hydrogenase. HydE, HydF and HydG are the [FeFe]-hydrogenase accessory proteins. For clarity, the Fe–S clusters of [FeFe]-hydrogenase have been omitted. The purple balls represent Ni or a Ni-containing centre in (a,b). The dark red balls represent the H-cluster in (c). ATP, adenosine triphosphate; AMP, adenosine monophosphate; GTP, guanosine triphosphate; GDP, guanosine diphosphate; PPi, pyrophosphate, Pi, phosphate; SAM, S-adenosyl methionine. When comparing LarA structure with all known folds using the VAST algorithm [33] , very few similarities with known structure could be identified (best score of 12.3 with E value of 1.45E−02, supplementary Table 8 ). Nevertheless, domain A was found to be weakly similar to the small domain of trimethylamine dehydrogenase, whose function is unknown [34] , and domain B was found to share some similarities with S -adenosyl methionine (SAM)-dependent methyltransferases [35] , although the SAM-binding site is neither conserved in the LarA structure nor in its primary sequence ( Fig. 3a and Supplementary Fig. 5 ). The catalytic site was predicted to be composed of 7 conserved residues (3 His, 2 Lys, 1 Asp and 1 Arg). XAS analyses suggest that at least two histidines are involved in Ni coordination. The conserved residues His108, His174 and His200 are good candidates for this function. A lactate molecule, showing the same O-C-C-O connectivity as glycerol and binding in a bidentate fashion, would also coordinate Ni. Finally, a yet undefined ligand would complete the coordination sphere, forming the predicted five coordinate square pyramidal site. Although nickel is absolutely required as a central component of the catalytic machinery of Ni-dependent enzymes, it can only be found in trace amounts in the environment. Therefore, sufficient nickel acquisition by these enzyme systems is a consequential process that can also be complicated by the expression of several nickel enzymes in the same organism [24] . Specific nickel-trafficking proteins are necessary to meet the distinct cellular demands for nickel. Those accessory proteins that are responsible for shuttling the nickel are thought to transfer nickel to the enzyme precursors through protein–protein interactions in a complex stepwise process [24] . However, Ni-binding accessory proteins were only identified in three of the eight Ni-dependent enzymes, that is, urease, [NiFe]-hydrogenase and carbon monoxide dehydrogenase [24] (illustrated for the urease at Fig. 8a ). In this study, we identified three new accessory proteins, LarB, LarC and LarE, which are required for the Lar activity. These accessory proteins participate in the incorporation of Ni in the Lar apoprotein, as their absence leads to an inactive Ni-less enzyme ( Fig. 6 ). In addition, this mechanism is flexible and conserved among Lars, as L. plantarum accessory proteins are able to activate the orthologous LarA Tt enzyme ( Table 1 ). Figure 8: Model of assembly of Lar metallocenter. ( a ) Assembly of urease metallocenter; one triangle represents one urease trimer of UreABC. UreD, UreE, UreF and UreG are the urease accessory proteins. ( b ) Proposed model for the assembly of Lar metallocenter. LarA is the Lar, while LarB, LarC and LarE are the Lar accessory proteins. ( c ) Assembly of [FeFe]-hydrogenase metallocenter. HydA is the [FeFe]-hydrogenase. HydE, HydF and HydG are the [FeFe]-hydrogenase accessory proteins. For clarity, the Fe–S clusters of [FeFe]-hydrogenase have been omitted. The purple balls represent Ni or a Ni-containing centre in ( a , b ). The dark red balls represent the H-cluster in ( c ). ATP, adenosine triphosphate; AMP, adenosine monophosphate; GTP, guanosine triphosphate; GDP, guanosine diphosphate; PPi, pyrophosphate, Pi, phosphate; SAM, S-adenosyl methionine. Full size image The incorporation of Ni in the apoprotein usually requires several accessory proteins and the hydrolysis of GTP ( Fig. 8a ). Yet, only one accessory protein, LarE, is required in the Lar system and ATP or GTP addition had no effect ( Supplementary Table 4 ). As LarE primary sequence shows similarities with ATP-utilizing enzymes of the PP-loop superfamily [4] , it is tempting to propose that the hydrolysis of ATP in AMP is taking place during the activation cascade, but more likely for the activation of LarE itself rather than for the activation of LarA. Furthermore, an excess of Ni can generally overcome the loss of one or several accessory proteins in other nickel-based systems [24] , whereas here Ni supplementation could neither complement the absence of any Lar accessory protein in vivo nor activate LarA apoprotein in vitro ( Fig. 1c and Supplementary Table 4 ). This suggests that the metallocenter of the Lar contains one or more ligand(s) in addition to Ni. In this case, LarE would serve as a scaffold protein for the synthesis of the Ni-containing metallocenter, which is then transferred into the catalytic site of LarA in one step. The synthesis of this metallocenter on LarE would require LarB and LarC. As LarC purified from L. lactis cells grown in the presence of Ni was shown to contain nickel independently of LarE and/or LarB, LarC is probably the Ni carrier of the Lar system (see Fig. 8b for a model). This activation mechanism is completely different from other maturase-activated Ni-dependent enzymes, where the assembly of the metallocenter takes place on the apoprotein and the Ni carrier transfers its Ni directly into the catalytic site ( Fig. 8a ). Yet, some similarities may be found with the activation mechanism described for [FeFe]-hydrogenases. This mechanism also involves one accessory protein (HydF), able to activate the apoprotein only when purified in presence of two other accessory proteins (HydG and HydE) [36] ( Fig. 8c ), but these similarities refer only to the overall sequence of the activation cascade. To conclude, this work reports the first molecular characterization of a Lar that is a novel maturase-activated Ni-dependent enzyme. The requirement for Ni is a novelty among racemases but the absence of an electron-withdrawing group on lactate may explain its use for the catalysis of lactate racemization by a postulated hydride transfer mechanism [17] . This hypothesis is supported by the identification of a similar catalytic mechanism in [NiFe]-hydrogenases [37] . In addition, the proposed assembly of the metallocenter on a single pre-activated maturation protein is novel and has not been described so far for any other maturase-activated Ni-dependent enzyme. Finally, the occurrence of the genes encoding the Lar maturation machinery in many bacterial and archaeal genomes containing or not a Lar-encoding gene shows the broad importance of this novel Ni-based system and also suggests that this machinery might have been recruited for another function probably linked with the activation of one or more Ni-dependent enzyme(s). Biological material and growth conditions Bacterial strains and plasmids used in the present study are listed in Supplementary Table 9 . All plasmid constructions were performed in Escherichia coli DH10B for pUC18Ery derivatives and in Lc. lactis NZ3900 for pNZ8048 derivatives. L. plantarum was grown in De Man–Rogosa–Sharpe (MRS) broth at 28 °C without shaking. Lc. lactis was grown in M17 broth supplemented with 0.5% glucose at 28 °C at 120 r.p.m. When appropriate, chloramphenicol and erythromycin were added to the media at 10 μg ml −1 and NiCl 2 at 1 mM concentration. For induction of Lar activity in L. plantarum , L-lactate sodium salt (Sigma-Aldrich, Belgium) was added at a concentration of 200 mM during the mid-log phase (OD 600 =0.6-0.7) and the cells were collected 4 h later. For the induction of genes under control of the nisA expression signals, Nisin A (Sigma-Aldrich, Belgium) was added during the early log phase (OD 600 =0.2-0.3) at a concentration of 1 mg l −1 and the cells were collected 4 h later. DNA techniques General molecular biology techniques were performed according to standard protocols [38] . Transformation of E. coli [39] , L. plantarum [40] and Lc. Lactis [41] was performed by electrotransformation. PCR amplifications were performed with the Phusion high-fidelity DNA polymerase (Finnzymes, Espoo, Finland). The primers used in this study were purchased from Eurogentec (Seraing, Belgium) and are listed in Supplementary Table 9 . Construction of the ΔlarOQ mutant The larQO deletion vector pGIR001 was constructed in two steps. Initially, a 1.62-kb fragment located downstream of larO was amplified by PCR with primers LP096A1 and LP099B3, digested with XbaI and KpnI, and cloned into similarly digested pUC18Ery. Subsequently, a 1.22-kb fragment comprising a fragment of larQ and lar ( MN ) was amplified by PCR with primers LP0102A3 and LP0101B1, digested with SpeI and XbaI, and inserted in the XbaI site of the plasmid obtained in the first step. The correct orientation of the insert was assessed by PCR with the primers LP096A1 and LP0101B1. This plasmid, pGIR001, harbours an in-frame fusion between the 5′ end of larO and a middle fragment of larQ . Since cloning of a DNA fragment containing larR seemed to be toxic to E. coli , the complete deletion of the lar ( MN ) QO operon could not be achieved. The pGIR001 suicide vector was used to delete larQO through a two-step homologous recombination process [40] . Deletion was carried out in L. plantarum NCIMB8826 (wild type), generating strain LR0001. The Δ larQO genotype was confirmed by PCR with primers LP096UP-3 and LP0105B1, located upstream and downstream of the recombination regions, respectively. Construction of Lc. lactis expression plasmids Plasmid pGIR100 was constructed by cloning of a DNA fragment comprising the whole larABCDE operon from L. plantarum NCIMB8826, which was amplified by PCR with primers StrepBZ_A2 and StrepB_B2, digested with PciI and SacI, and then ligated in the pNZ8048 plasmid digested with NcoI and SacI. The resulting plasmid was transformed in Lc. lactis . Plasmids bearing deleted versions of the larA–E operon for expression in Lc. lactis were all derived from pGIR100: pGIR200 (Δ larA ), pGIR300 (Δ larB ), pGIR500 (Δ larC ), pGIR600 (Δ larD ) and pGIR700 (Δ larE ). For each construction, pGIR100 was first methylated with Dam methylase and S-adenosyl methionine (New England Biolabs). PCR amplification was performed in order to obtain a fragment comprising the whole pGIR100 plasmid, deleted of the gene of interest, using primers LarZ-X_A and LarZ-X_B (X stands for the gene to be deleted), digested with ClaI and self-ligated, generating an in-frame deletion of the selected gene. The ligation mixture was digested with DpnI before transformation in Lc. lactis in order to digest the original pGIR100 plasmid used as template. The plasmid sequences were confirmed by sequencing with primers UP_PNZ8048′ and 632SEQA4 to 632SEQA14. Construction of plasmids for the purification of Lar proteins Plasmids for expression of selected StrepII-tagged Lar proteins together with expression of all other Lar proteins were derived from pGIR100 (containing the entire larA–E operon): pGIR112 (LarA-Strep-tag), pGIR122 (LarB-Strep-tag), pGIR131 (Strep-tag-LarC) and pGIR172 (LarE-Strep-tag). A fragment comprising the whole pGIR100 plasmid was amplified by PCR using primer pairs LarStrep_A/LarStrep_B for pGIR112, BT_A/BT_B for pGIR122, TC_A/TC_B for pGIR131 and LarE_TA/LarE_TB for pGIR172. In every case, one of the two primers contained the sequence encoding a StrepII-tag either in the upstream or the downstream primer ( Supplementary Table 9 ). Amplified DNA fragments were digested with NheI and self-ligated, generating a 30-bp in-frame insertion of a fragment containing the StrepII-tag at the desired position (either 5′ or 3′ of the targeted gene). The ligation mixture was digested with DpnI before transformation in Lc. lactis in order to digest the original pGIR100 plasmid used as template. The sequence of the expression cassettes was verified by sequencing with primers UP_PNZ8048′ and 632SEQA4 to 632SEQA14. Plasmid pGIR012 (LarA-Strep-tag alone) was obtained by PCR amplification of pGIR112 with primers LarE_TA and LarStrep_B, NheI digestion, self-ligation and transformation in Lc. lactis . Plasmid pGIR022 (LarB-Strep-tag alone) was obtained by PCR amplification of pGIR122 with primers LarB_A and LarBT_B, digestion with NcoI and HindIII, insertion in a similarly digested pNZ8048 by ligation and transformation in Lc. lactis . Plasmid pGIR031 (Strep-tag-LarC alone) was obtained by PCR amplification of pGIR131 with primers Pci1Tag_A and LarC_B, digestion with PciI and HindIII, insertion in a NcoI and HindIII digested pNZ8048 by ligation and transformation in Lc. lactis . Plasmid pGIR072 (LarE-Strep-tag alone) was obtained by PCR amplification of pGIR172 with primers LarE_A and StrepP_B, NcoI digestion, self-ligation and transformation in Lc. lactis . Plasmid pGIR182 (LarA Tt -Strep-tag in the presence of L. plantarum maturases) was obtained by cloning a fragment containing larA Tt amplified by PCR from genomic DNA of T. thermosaccharolyticum with primers LarA_Th_A and LarA_Th_B and digested by NcoI and NheI. This fragment was ligated with a fragment of pGIR112 amplified by PCR with primers LarStrep_A and LarA_Th_C and digested by PciI and NheI. The ligation mixture was then restricted by BamHI to digest plasmid pGIR112 and transformed in Lc. lactis . Plasmid pGIR082 (LarA Tt -Strep-tag alone) was obtained by PCR amplification of pGIR182 with primers LarA_Th_A and LarA_Th_B2, digestion with NcoI and KpnI, and insertion in a similarly digested pNZ8048 by ligation. In all cases, the sequence of the expression cassettes was verified by sequencing. Construction of plasmids for the modification of LarC The intermediate plasmid pGEM_larABCDE was constructed by subcloning of a DNA fragment comprising the whole larABCDE operon from L. plantarum NCIMB8826, which was amplified by PCR with primers StrepBZ_A2 and StrepB_B2 and ligated into the pGEM-T Easy (Promega) [42] . The intermediate plasmids pGEM_larABC1ΔC2DE and pGEM_larABC-fusedDE were derived from the intermediate plasmid pGEM_larABCDE (containing the entire larA–E operon). PCR amplification were performed in order to obtain a fragment comprising the whole pGEM_LarABCDE plasmid, deleted of larC2 , and a fragment comprising the whole pGEM_LarABCDE plasmid, with a 1 bp insertion at the end of larC1 , using primers LarZ-C2b_A and LarZ-C2b_B and primers pG_LarCC_A and LarCC_B, respectively. The PCR fragments were digested with BstB1 and self-ligated. The ligation mixtures were digested with DpnI before transformation in E. coli DH10B in order to digest the original pGEM_larABCDE plasmid used as template and purified from E. coli DH10B (Dam + ). Plasmid pGIR400 (Δ larC2 ) and pGIR150 (LarC-fused) were constructed by cloning of a DNA fragment comprising the whole larABC1 Δ C2DE operon or larABC-fusedDE operon, which was obtained by digestion of pGEM_larABC1ΔC2DE or pGEM_larABC-fusedDE with PciI and SacI, and ligated in the pNZ8048 plasmid digested with NcoI and SacI. The resulting plasmids were transformed in Lc. lactis . Plasmid pGIR151 (Strep-tag-LarC-fused) was derived from plasmid pGIR150 (LarC-fused) as described for plasmid pGIR131 (Strep-tag-LarC). Plasmid pGIR051 (Strep-tag-LarC-fused alone) was derived from plasmid pGIR151 (Strep-tag-LarC-fused) as described for plasmid pGIR031 (Strep-tag-LarC alone). The plasmid sequences were confirmed by sequencing with primers UP_PNZ8048′ and 632SEQA4 to 632SEQA14. Microarray experiments A culture of L. plantarum TF101 (Δ ldhL ) [43] was grown to an OD 600 of 0.75 and then divided into three sub-cultures. Pure L-lactate (200 mM final concentration) was added to one of the sub-cultures. An equimolar mixture of D- and L-lactate (100 mM final concentration for each isomer) was added to a second sub-culture. The third subculture was not treated. The three sub-cultures were further incubated for 90 min, before harvesting by centrifugation (5,000 g , 10 min). Cell pellets were stored at −20 °C until RNA extraction. Cells were disrupted with four subsequent 40-s treatments in a Fastprep cell disrupter, interspaced by 1 min on ice (Qbiogene Inc., Illkirch, France) [44] . After disruption, RNA was isolated with a High Pure RNA Isolation Kit, which included 1 h of treatment with DNase I (Roche Diagnostics, Mannheim, Germany) [44] . The RNA quality was assessed using the RNA 6000 Nano Assay in an Agilent 2100 Bioanalyzer (Agilent technologies, Palo Alto, CA, USA) following the manufacturer’s instructions. cDNA synthesis was carried out by the CyScribe Post-Labelling and Purification kit (Amersham Biosciences, Buckinghamshire, UK) following the manufacturer’s instructions. Hybridization was performed on custom designed L. plantarum WCFS1 11 K Agilent oligo microarrays using the Agilent hybridization protocol (version 5.5). These microarrays contained an average of three probes per gene. The hybridization scheme contained the following cDNA comparisons: (a) untreated culture versus L-lactate-treated culture and (b) untreated culture versus DL-lactate-treated culture. Slides were scanned with an Agilent Scanner G2565AA and the intensity of the fluorescent images was quantified using Agilent Feature Extraction software (version A.7.5). Data were extracted, corrected for background and normalized using the LOWESS algorithm in BASE [44] . The normalized transcriptome data have been deposited in the Gene Expression Omnibus (GEO) database under accession code GSE43518. First, significantly regulated probes were selected based on a fold change (Cy5/Cy3 intensities) higher than 4.0 or lower than 0.25. Genes for which >50% of the probes were not significantly regulated were considered as not regulated. For the remaining genes, the fold change of gene expression was calculated as the average of the fold change between significantly regulated probes. Protein extraction and analysis Cells from a 50-ml culture of Lc. lactis or L. plantarum were collected by centrifugation at 5,000 g for 10 min and washed twice with 25 ml of 60 mM Tris-maleate buffer at pH 6.0 (TM buffer). Cells were resuspended in 0.5 ml TM buffer and transferred to a 2-ml microtube containing 0.5 ml of a suspension of 0.17–0.18 mm glass beads (Sartorius Mechatronics, Belgium) in TM buffer. Lysis was performed by running the microtubes two times for 1 min at 6.5 m s −1 in a FastPrep-24 (MP, Belgium). Microtubes were cooled for 5 min on ice between the runs. After lysis, the soluble fraction (referred to as the crude extract) was collected by centrifugation at 13,000 g for 15 min (4 °C). When larger volumes of culture were used, cells were resuspended and lysed in 50-ml Falcon tubes (BD, NJ, USA) using the same protocol. Routine protein content was measured with the Bradford assay [45] . Since the Bradford assay is highly variable from one protein to another, the NanoOrange protein quantification kit (Invitrogen) was used for a lower protein-to-protein variability [46] . The conversion from g l −1 to mol l −1 was calculated with the theoretical molecular weight of the proteins, assuming they were 100% pure. The weight ratio of LarC1/LarC was estimated to be 1.5/1, yielding a molecular ratio of 2.4/1. Sodium dodecyl sulphate polyacrylamide gel electrophoresis (SDS-PAGE) was performed with 10% acrylamide gels [47] . The proteins were stained with Coomassie Brilliant Blue R and the protein mass ladder used was the PageRuler Prestained Protein Ladder (Fermentas, France). For protein identification, the protein band was cut off the gel, digested and analysed on an Applied Biosystems 4800 MALDI TOF/TOF Analyser [48] . The MALDI-TOF data have been deposited in the PRoteomics IDEntifications (PRIDE) database under accession code PXD000775. Protein purification Affinity chromatography was performed with Gravity flow Strep-Tactin Superflow high capacity columns of 1 ml or 5 ml (ref. 49 ), with the following adaptations. For 1 ml column purification, 1 l of Lc. Lactis culture was washed and cells were lysed as described above in buffer W (100 mM Tris-HCl, 150 mM NaCl, pH 7.5) instead of TM buffer. The column, equilibrated with 2 ml buffer W, was loaded with up to 10 ml crude extract, washed six times with 1 ml buffer W, and eluted 10 times with 0.5 ml buffer E (buffer W+2.5 mM desthiobiotin). The following adaptations were made for the Lar proteins: LarA, 60 mM Tris-Maleate at pH 6 was used as lysis buffer and the crude extract was equilibrated at pH 7.5 (using 500 mM Tris at pH 10) before loading; LarB, Triton X-100 (0.1% v / v ) was added to all buffers; LarE, 300 mM NaCl instead of 150 mM was used in all buffers. For purifications with 5 ml columns, all volumes were increased fivefold. In order to purify the Lar proteins to homogeneity (for crystallization purposes only), a second step of purification was performed using size exclusion chromatography. A Hiload 26/60 superdex 200 prep grade resin (Amersham Pharmacia Biotech) was used with 50 mM MES at pH 6.0 and 150 mM NaCl as an elution buffer (300 mM NaCl for LarE). Before protein loading, the sample was concentrated using a Centricon Plus-70 centrifugal (30 kDa cut-off) filter unit (Merck Millipore, Germany). After collection of the fractions containing the target protein, as determined by absorbance at 280 nm, samples were concentrated again using an Amicon Ultra-4 (10 kDa cutoff) centrifugal filter (Merck Millipore, Germany). The purified Lar proteins were stored at −80 °C in the elution buffer supplemented with glycerol to 20% of the final volume. The Lar activity of LarA was stable for several weeks in this condition. Lar activity The Lar activity was assayed by measurement of the D- to L-lactate or L- to D-lactate conversion. Cell extracts or purified proteins were incubated at the appropriate dilution with 20 mM D- or L-lactate in 60 mM MES buffer (pH 6) at 35 °C (LarA Lp ) or 50 °C (LarA Tt ) for 10 min. A dilution factor of 10 and 50 was used for L. plantarum and Lc. Lactis cell extracts, respectively. The reaction was stopped by incubating the reaction mixture for 10 min at 90 °C. The lactate conversion was measured by enzymatic lactate oxidation into pyruvate using a D-lactic acid/L-lactic acid commercial test (R-Biopharm, Germany). The protocol was adapted to 100 μl reaction volumes in 96-well half-area microplates (Greiner, Alphen a/d Rjin, theNetherlands). The NADH absorbance was read at 340 nm with a Varioskan Flash (Thermo Scientific). One unit of Lar activity is defined as the amount of enzyme required to convert 1 μmol of lactate in 1 min. For kinetics measurements, a substrate concentration ranging from 5–320 (or 400) mM was used. The K m and k cat were calculated by non-linear regression using the Michaelis–Menten equation. For time-dependent LarA inactivation assays, 25 pmol of purified LarA Lp was incubated at room temperature in a 100 μl solution containing 60 mM MES buffer (pH 6) supplemented with NiCl 2 (10 mM) or L-ascorbic acid (10 mM). Samples (10 μl) were removed every 10 min for 80 min for measuring Lar activity with L-lactate as substrate. Nickel assays For Ni quantification by ICP-AES, the sample was first mineralized. A solution of 0.5 ml H 2 O 2 and 0.5 ml of HNO 3 (Merck Millipore, Germany) was added to 1 ml of protein sample and the mixture was then heated to dryness on a heating plate. The residues were solubilized with 0.5 ml of HNO 3 and diluted to 10 ml with H 2 O. The elements were measured by ICP-AES on an ICAP 6500 (Thermo Scientific). For Ni quantification using PAR, the protein sample was denatured for 10 min at 90 °C before incubation at room temperature with 100 μM PAR in 100 mM Tris-HCl buffer at pH 7.5 for 2 min. The absorbance was read from 300 nm to 600 nm by steps of 2 nm to confirm that the visible spectrum corresponds with the expected PAR-Ni spectrum [22] . For Ni quantification, the absorbance was read at 496 nm. To quantify Ni leakage from LarA by the PAR assay, 1.5 nmol of LarA Lp was used and the absorbance (496 nm) was monitored every minute for 80 min. In vitro LarA activation assays The effect of accessory Lar proteins and cofactors on the in vitro activation of LarA NiΔBCE (apo-LarA) by LarE NiBC was assessed by incubating 2 pmol of LarA NiΔBCE at room temperature in a 50-μl solution of 60 mM MES buffer (pH 6) supplemented with 20 pmol LarB, larC or LarE and various cofactors (NiCl 2 , adenosine triphosphate, guanosine triphosphate, cysteine, S-adenosyl methionine, potassium hydrogen carbonate, coenzyme A, nicotinamide adenine dinucleotide and thiamine diphosphate), when required. Lar activity was measured by sampling 10 μl of the solution at 0, 30, 60 and 120 min. For assessing the activation potential of the different forms of LarE (LarE NiBC , LarE BC or LarE NiΔBC ), 1.4 pmol of LarA NiΔBCE was mixed with 280 pmol of LarE. Crystallization and structure determination of LarA For initial screening experiments, a LarA Tt solution at a concentration of 16 mg ml −1 0.5 mM MES at pH 6.0 and 1.5 mM NaCl was submitted to the high-throughput crystallization facility at EMBL Hamburg [50] using the sitting drop vapour diffusion setup. After optimization of the best results, two different crystal forms were obtained in hanging drop experiments. The first form was obtained at 18 °C from a reservoir containing 22% polyethylene glycol monomethyl ether 5000, 0.2 M ammonium sulphate, 0.1 M MES pH 6.5, 0.2 M sodium malonate (pH 7.0) and 0.02% ( w / v ) sodium azide. The hanging drop was formed by mixing 2 μl of the protein solution with 2 μl of the reservoir solution. These crystals that appeared after a few days were trigonal, of the space group P3 1 21 or P3 2 21, with a =227 Å and c =48 Å, but they diffracted very poorly (~4 Å resolution) with very diffuse spots and they could not be used for crystal structure analysis. A second crystal form was obtained in very similar conditions: the only difference was the replacement of sodium malonate with 3% ( v / v ) ethylene glycol in the reservoir solution. These crystals appeared after about 2 months, they belong to the orthorhombic system and diffracted to much higher resolution and were used for crystal structure analysis. All data were collected at ESRF on beamline BM30A. A native data set was collected after soaking a crystal for a few seconds in a solution similar to the mother liquor but containing 20% ( v / v ) ethylene glycol as a cryoprotectant and flash-cooled at 100 K. A mercury derivative was obtained by soaking a crystal for 48 h in the same solution containing also 1 mM HgCH 3 Cl and was used for MAD data collection at three wavelengths. This mercury derivative was not isomorphous with the native data. All the data sets were processed and scaled using the XDS programme package [51] . The structure was solved by the MAD method applied to the mercury derivative using the Auto-Rickshaw procedure [52] . A substructure containing four heavy atoms was successfully solved by SHELXD [53] . The initial phases and molecular model were obtained from SHELXE [54] and they were further improved in the Auto-Rickshaw pipeline using PHASER [55] , MLPHARE, PIRATE, REFMAC5 (ref. 56 ) from the CCP4 suite [57] , RESOLVE [58] and ARP_wARP [59] . A total of 226 residues in three fragments were finally docked in the sequence. Surprisingly, all these residues belonged to the same protein chain. This model was used for molecular replacement in the native data set and PHASER [55] succeeded to locate two copies in the asymmetric unit. Many cycles of model building in ARP_wARP [59] allowed to build large parts of the two chains. The model was manually completed using COOT [60] and refined with REFMAC5 (ref. 56 ). Electron density did not appear for residues 30–36 and for about 10 residues in the C-terminal part of the two chains. The final model contains 588 water molecules, 5 sulphate ions, 1 ethylene glycol molecule and 1 supposed Mg 2+ ion located on the non-crystallographic two-fold axis linking the two protein chains. Atomic coordinates for the LarA of T. thermosaccharolyticum have been deposited in the RSCB Protein Data Bank (PDB) database under accession code 2YJG. EXAFS and XANES analyses Protein samples from Lc. lactis . LarA Tt (4.5 mM, 0.1 mol Ni per mol protein) and LarA Lp (1.2 mM, 0.17 mol Ni per mol protein) were prepared in 10 mM Tris-HCl (pH 7.5), 20% glycerol buffers for XAS. Samples were kept at −80 °C and transported at liquid nitrogen temperatures until run. X-ray absorption data collection was carried out at SSRL (Stanford Synchrotron Radiation Lightsource, 3 GeV ring) beam line 7-3 equipped with a 13-element Ge detector array with a Si(220) phi=0° double crystal monochromator and a liquid helium cryostat for the sample chamber. Söller slits were used to reduce scattering and a 3-μm Z-1 element filter was placed between the sample and the detector. Internal energy calibration was performed by collecting spectra simultaneously in transition mode on a nickel metal foil. Data averaging and energy calibration was performed using SixPack [61] . The first inflection points from the XANES spectral regions were set to 8,331.6 eV for nickel foil. The AUTOBK algorithm available in the Athena software package was employed for data reduction and normalization [62] . A linear pre-edge function followed by a quadratic polynomial for the post-edge was used for background subtraction followed by normalization of the edge-jump to 1. EXAFS data was extracted using an R bkg of 1, and a spline from k =1–14 Å −1 with no clamps. The k 3 -weighted data were fit in R-space over the k =2–12.5 Å −1 region with E 0 for nickel set to 8,340 eV. All data sets were processed using a Kaiser–Bessel window with a d k =2 (window sill). Artemis employing the FEFF6 and IFEFFIT algorithms was used to generate and fit scattering paths to data [62] , [63] , [64] . Single scatter and multiple scatter fits were performed as described below. Average values and bond lengths obtained from crystallographic data were used to construct initial fitting models for multiple scatter analysis [65] . The paths from a particular multiple scattering model were generally afforded two degrees of freedom and were fit in terms of the distance from the first ligand atom–metal bond and a ligand-specific sigma square component of the Debye–Waller factor [66] , [67] , [68] . To assess the goodness of fit from different fitting models, the goodness of fit (% R ), χ 2 , and reduced χ 2 ( χ ν 2 ) were minimized. Increasing the number of adjustable parameters is generally expected to improve the % R ; however χ ν 2 may go through a minimum then increase indicating the model is over-fitting the data. Bioinformatic analyses of Lar proteins To identify conserved residues in LarA proteins, 148 LarA homologues were aligned with clustalX2 (ref. 69 ), and a phylogenetic tree was constructed using the neighbour-joining method [70] . Out of these, 10 homologues selected to represent the diversity of LarA proteins were aligned with clustalX2 (ref. 69 ). To study the distribution and clustering of Lar proteins among bacterial and archaeal genomes, BlastP searches were performed using L. plantarum Lar protein sequences of strain WCFS1 (a single colony isolate of NCIMB8826) as queries against all complete prokaryotic genomes of the NCBI database (release 187). BlastP searches were performed using default parameters with a cutoff E-value of 10 −5 in order to only select proteins that show a high similarity with Lar proteins. For LarA homologues, proteins were excluded when their length were <90% or >130% compared with the length of LarA Lp . When several genomes of the same species were available, the genome containing the highest content in lar genes was retained. Gene clusters based on gene identification numbers were assessed by considering all lar genes as belonging to the same cluster when there was a maximum of one gene between them on the chromosome. Since >500 homologues were found for LarD due to the high similarity level of members of the aquaglyceroporin family, only 9 homologues present in lar operons were retained as true LarD. Since some larC genes contain a frameshift, this led to the misleading annotation of some larC homologues as pseudogenes that were overlooked by the BlastP programme. Some of them were identified manually by looking at the flanking regions of lar genes, but others may still remain undetected. Accession codes: Normalized transcriptomic data have been deposited in the GEO database under accession code GSE43518. Atomic coordinates for the LarA of T. thermosaccharolyticum have been deposited in the PDB database under accession code 2YJG. The MALDI-TOF data have been deposited in the PRIDE database under accession code PXD000775 . How to cite this article: Desguin, B. et al. Lactate racemase is a nickel-dependent enzyme activated by a widespread maturation system. Nat. Commun. 5:3615 doi: 10.1038/ncomms4615 (2014).